Effects of electronegative substitution on the optical and electronic properties of acenes and diazaacenes Large acenes, particularly pentacenes, are important in organic electronics applications such as thin-film transistors. Derivatives where CH units are substituted by sp 2 nitrogen atoms are rare but of potential interest as charge-transport materials. In this article, we show that pyrazine units embedded in tetracenes and pentacenes allow for additional electronegative substituents to induce unexpected redshifts in the optical transitions of diazaacenes. The presence of the pyrazine group is critical for this effect. The decrease in transition energy in the halogenated diazaacenes is due to a disproportionate lack of stabilization of the HOMO on halogen substitution. The effect results from the unsymmetrical distribution of the HOMO, which shows decreased orbital coefficients on the ring bearing chlorine substituents. The more strongly electron-accepting cyano group is predicted to shift the transitions of diazaacenes even further to the red. Electronegative substitution impacts the electronic properties of diazaacenes to a much greater degree than expected. The larger acene cores provide a particularly attractive framework for the design of molecules with tunable properties that can be useful for organic electronic applications. Pentacenes such as 1 [1] or 5 , but also 2 (first prepared by Hinsberg [2] ), are of major interest as hole-transport materials in thin-film transistors [3] and have high charge-carrier mobilities, because of their favourable solid-state packing and small reorganization energies [4] , [5] , [6] ; pentacene is also a component of reference for systems in the development of small-molecule organic solar cells [7] . Although Houk suggested that larger N -heteroacenes could behave as electron-transport materials when suitably substituted [8] , to date acenes have generally functioned as hole-transport materials. Only a few acenes have shown appreciable electron mobilities [9] , [10] , [11] , [12] . To realize the full potential of acenes and heteroacenes, it is essential to expand the scope of materials available. 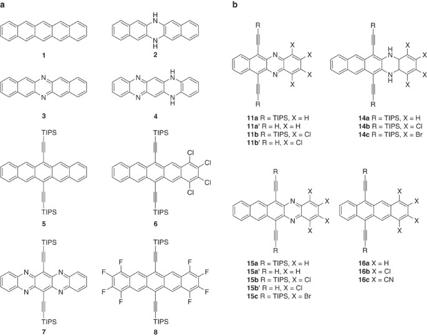Figure 1: Pentacene compounds of current and historical interest and the target compounds produced herein. (a) Compounds prepared by (1) Clar,1(2) Hinsberg2, (3) Zimmermann22; (4) Fischer30, (5) Anthony5; (6) Bao15, (7) Bunz13, (8) Bao10. (b) Compounds prepared in this paper (11a,b,14a–c,15a–c) and calculated model compounds (11a′,b′,15a′,b′,16a–c). Figure 1a shows recent and historical members in the series of pentacenes [13] , [14] . Chlorinated pentacenes such as 6 were processed into ambipolar transistors. Chlorination lowers both HOMO and LUMO, but with the former effect insufficient to preclude hole injection, whereas the latter effect facilitates electron injection; however, the optical gap does not change to any appreciable extent [15] . The tetrachloro substitution only led to a slight shift in the absorption maximum going from 643 nm for 5 [16] to 654 nm for 6 in solution, suggesting that chlorine substitution had comparable impact on both the ground and first excited states [17] , [18] , [19] . Lowering the absorption energies can be useful in the context of organic solar cells when looking for acene derivatives showing absorption into the near-infrared, as observed in Anthony's hexacenes and heptacenes [20] , [21] . Figure 1: Pentacene compounds of current and historical interest and the target compounds produced herein. ( a ) Compounds prepared by ( 1 ) Clar, [1] ( 2 ) Hinsberg [2] , ( 3 ) Zimmermann [22] ; ( 4 ) Fischer [30] , ( 5 ) Anthony [5] ; ( 6 ) Bao [15] , ( 7 ) Bunz [13] , ( 8 ) Bao [10] . ( b ) Compounds prepared in this paper ( 11a,b , 14a–c , 15a–c ) and calculated model compounds ( 11a′,b′ , 15a′,b′ , 16a–c ). Full size image We report here the simple synthesis of novel heteroacenes, viz . diazapentacene 15a , the halogenated diazatetracene 11b and the tetrahalodiazapentacenes 15b,c ( Fig. 1b ). Electronegative substitution, that is, transforming 11a→ 11b and 15a → 15b,c , causes surprising bathochromic shifts in absorption, in addition to the improved reducibility anticipated through stabilization of the LUMOs by electronegative substitution [22] . Synthesis Condensation of 9 ( Fig. 2a ) with 10b gave tetrachlorodiazatetracene 11b smoothly and in good yields. For comparison purposes we also re-synthesized 11a [23] . The diamine 13 ( Fig. 2b ) was obtained by LiAlH 4 reduction of 12 (ref. 24 ) and reacted with 10a–c to furnish the N,N -dihydrodiazapentacenes 14a–c in moderate yields; 14a–c were oxidized by manganese dioxide to give 15a–c after chromatography as green-black, environmentally stable crystalline materials almost quantitatively. 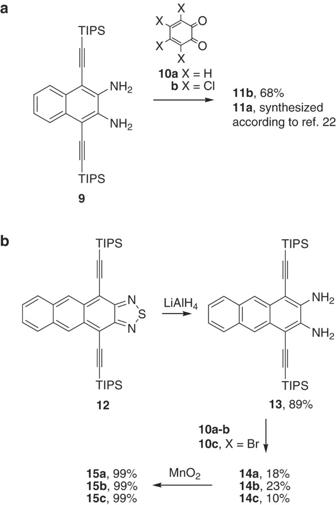Figure 2: Synthesis of diazatetracene11band diazapentacenes15. (a) The condensation of the diamine9with theortho-quinones10aand10bfurnished the diazaacenes11aand11bin excellent yield. (b) On reacting13with10, the NH intermediates14a–care isolated and oxidized efficiently to15a–c, respectively, by manganese dioxide. Figure 2: Synthesis of diazatetracene 11b and diazapentacenes 15 . ( a ) The condensation of the diamine 9 with the ortho -quinones 10a and 10b furnished the diazaacenes 11a and 11b in excellent yield. ( b ) On reacting 13 with 10 , the NH intermediates 14a–c are isolated and oxidized efficiently to 15a–c , respectively, by manganese dioxide. 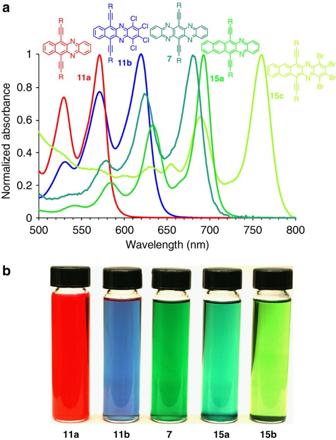Figure 3: UV-Vis spectra of selected heteroacenes. (a) Long-wavelength normalized UV-Vis spectra in hexane; R=TIPS in all cases. (b) Photograph of solutions of heteroacenes in hexane. The combined effects of annulation and halogenation lead to a shift of absorption from 571 to 758 nm. The spectrum of15bis almost superimposable onto that of15c. The halo-substitution in both tetracenes and in pentacenes leads to significant redshifts in absorption. Chlorine and bromine substituents are equally effective. The UV-Vis spectrum of7was taken from Miaoet al.13 Full size image Optical spectra and cyclic voltammetry Figure 3a shows the long-wavelength features of the UV-Vis spectra of a selection of the diazatetracenes and diazapentacenes and, as a comparison, the UV-Vis spectrum of the tetraazapentacene 7 (ref. 13 ). Figure 3b shows a photograph of solutions of these materials. The absorption spectrum of 11b (in hexane) shows a λ max of 617 nm, whereas 11a , the parent, shows a λ max of 571 nm; that is, the tetrachloro substitution leads to a redshift of 1,306 cm −1 or 0.16 eV, whereas, in comparison, tetrachloropentacene 6 shows an absorption maximum only 0.032 eV lower in energy than that of the parent compound 5 , according to reported UV-Vis spectra (ref. 24 ). Figure 3: UV-Vis spectra of selected heteroacenes. ( a ) Long-wavelength normalized UV-Vis spectra in hexane; R=TIPS in all cases. ( b ) Photograph of solutions of heteroacenes in hexane. The combined effects of annulation and halogenation lead to a shift of absorption from 571 to 758 nm. The spectrum of 15b is almost superimposable onto that of 15c . The halo-substitution in both tetracenes and in pentacenes leads to significant redshifts in absorption. Chlorine and bromine substituents are equally effective. The UV-Vis spectrum of 7 was taken from Miao et al. [13] Full size image The UV-Vis spectra of the NH compounds 14a–c are similar to each other, but show a slight hypsochromic, rather than bathochromic, shift when going from the parent to the halogenated species ( 14a : λ max =493 nm; 14b : λ max =479 nm; 14c : λ max =482 nm ( Supplementary Figs S1 and S2 ), whereas 15a–c again show bathochromically shifted spectral features. Table 1 shows parameters characterizing the absorption spectra, the results of the cyclic voltammetry measurements ( Supplementary Table S1 ) and of quantum chemical calculations using density functional (DFT) and time-dependent density functional theory (TD-DFT) of derivatives of 11 and 15 ( Supplementary Table S2 ). Table 1 Absorption and emission maxima and electrochemistry of the investigated heteroacenes. Full size table The diazapentacene 15a has a molar extinction coefficient ( =1.9 × 10 4 ; Table 1 ) that is close to that of 5 ( =2.0 × 10 4 ). The introduction of halogen substituents in 11 and 15 leads to some ( 11→ 11b , 15a → 15b ) decreases in the extinction coefficients. Also the redshifts observed in the solution absorption persist in the solid state and are approximately 800–900 cm −1 when going from solution into the solid state for the diazapentacenes ( Table 1 ). Both of the tetracenes ( 11a and 11b ), as well as diazapentacene 15a , are fluorescent, the diazatetracenes more so than the diazapentacenes, whereas the halogenated diazapentacenes are non-fluorescent. Quantum chemical calculations To further explore the effect of electronegative substitution in heteroacenes, we performed DFT and TD-DFT calculations on model compounds with structures derived from 11 and 16 . Table 1 shows the TD-DFT values of the vertical transition energies ( S 1 vert ) for the lowest-lying singlet excited states of model compounds 11a′ , 11b′ , 15a′ and 15b′ . The calculations reproduce the trends observed in the experimental data of 11a,b and 15a,b ; TD-DFT calculations for the tetracenes 16a and 16b predict only a very small redshift in absorption as a result of chlorination, which is also consistent with experimental data for the corresponding homolog pentacenes, 5 and 6 . 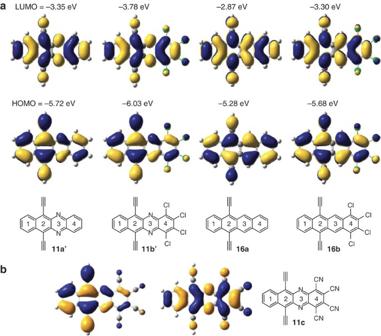Figure 4: Frontier molecular orbitals of acene derivatives. HOMO, middle; LUMO, top. The middle bottom row shows the structural formulae and numbering of the rings. (a) The LUMOs of the four compounds are very similar to each other. Both the LUMOs of11b′and16bexperience a stabilization of 0.43 eV through the chlorine substitution. The HOMOs of11a′/11b′ and16a/16bresemble each other qualitatively but are pair wise (11/16) different. The differences are pronounced in the rings 3 and 4 as particularly in the HOMO of11a′the orbital coefficients (see SI) on the rings 3 and 4 are small; as a consequence the chlorine substituents are less effective in stabilizing the HOMO (going from11a′to11b′), mirroring the optical behaviour seen in compound11b. (b) Frontier molecular orbitals (HOMO 6.30 eV, left; LUMO 4.49 eV, right; gap=1.81 eV) of tetracyanodiazaacene11c. Calculated by DFT using B3LYP/6-311+G* basis sets. Compared to11a′ calculated on the same level of theory, the optical band gap (S0–S1transition) shrinks from 2.07 to 1.38 eV. Figure 4a shows the frontier molecular orbitals (energy in eV) of 11a′ / 11b′ and 16a / 16b . In both pairs, stabilization of the LUMOs results when attaching four chlorine substituents. The stabilization is 0.43 eV in both 11b′ and 16b . More importantly, on going from 11a′ to 11b′ the HOMO is only stabilized by 0.31 eV, whereas in the case of 16a/16b the HOMO stabilization is 0.40 eV, very similar to that observed for the LUMO. On the basis of computational results, the contribution (sum of the squared orbital coefficients) from rings 3 and 4 is about three times as large in 16a as in the heteroacene 11a′ . To investigate the influence of even stronger acceptors, we performed quantum chemical calculations on model 11c ( Fig. 4b ). The HOMO of 11c is predominantly localized on rings 1 and 2, whereas the LUMO is extended over all four rings; as a result, the calculated optical gap shrinks from 2.07 eV in 11a to 1.38 eV in 11c . Figure 4: Frontier molecular orbitals of acene derivatives. HOMO, middle; LUMO, top. The middle bottom row shows the structural formulae and numbering of the rings. ( a ) The LUMOs of the four compounds are very similar to each other. Both the LUMOs of 11b′ and 16b experience a stabilization of 0.43 eV through the chlorine substitution. The HOMOs of 11a ′/ 11b ′ and 16a/16b resemble each other qualitatively but are pair wise ( 11/16 ) different. The differences are pronounced in the rings 3 and 4 as particularly in the HOMO of 11a′ the orbital coefficients (see SI) on the rings 3 and 4 are small; as a consequence the chlorine substituents are less effective in stabilizing the HOMO (going from 11a′ to 11b′ ), mirroring the optical behaviour seen in compound 11b . ( b ) Frontier molecular orbitals (HOMO 6.30 eV, left; LUMO 4.49 eV, right; gap=1.81 eV) of tetracyanodiazaacene 11c . Calculated by DFT using B3LYP/6-311+G* basis sets. Compared to 11a ′ calculated on the same level of theory, the optical band gap (S 0 –S 1 transition) shrinks from 2.07 to 1.38 eV. Full size image Larger functionalized heteroacenes are virtually unknown. The synthesis of the diazatetracenes 11a,b proceeds smoothly by simple condensation of a diamine with an ortho -quinone. In the case of the diazapentacenes 15a–c , the condensation first leads to 14a–c , which are then oxidized into 15a–c . It has been noted that the formally anti-aromatic 14a–c [1] , [25] are stabilized by the interplay of energetically advantageous enamine groups and the presence of two Clar sextets instead of one for the heteroacenes 15a-c . In the diazatetracenes 11 , this delicate energetic balance is such that the overall aromaticity drives the formation of 11 , and the significantly more anti-aromatic NH compounds are not observed as already shown by Hinsberg for the parent diazatetracene in 1901 (refs 2 , 25 ). However, oxidation of 14 into 15 is facile and quantitative. The most interesting and important discovery of this contribution is the significant redshifts that are observed when attaching halogen substituents to diazaacenes. The spectral redshift observed when going from 11a to 11b and from 15a to 15b or 15c is evident in Figure 3 . By change of substituent and size of the acene framework, an absorption range from 561 to 758 nm can be 'tuned in' in 11 and 15 . The expected acene-type vibronic fine structure is observed for all of the compounds and, although the extinction coefficient decreases on addition of the electronegative substituents, the effect is not dramatic, suggesting that these materials could be useful absorbers. Electronegative substitution on π systems can lead to either blue- or redshifted or almost unchanged absorption spectra; chlorination, for example, induces bathochromic shifts in 9,10-dichloroanthracene [17] and in some chlorinated nitro-aminodiazobenzene derivatives of disperse red [18] . Such electronegativity effects occur if either the HOMO or the LUMO is particularly stabilized or not; they are especially pronounced in molecules with disjoint orbital structures, where HOMO and LUMO are localized on different parts of the molecule. However, the contrast of the pairs 11a→ b / 15a → b and 5/6 was unusually large and unanticipated. Also surprisingly, the effect of bromine and chlorine substituents on the optical features of the diazaacenes is almost identical. This is however consistent with the similar inductive and mesomeric properties of these two halogens (Br: F =+0.45, R =–0.22; Cl: F =+0.42, R =–0.19; F =field effect parameter, R =resonance parameter) that is, both substituents function as moderately inductive ( σ ) electron-withdrawing groups and as weak π -donors, as indicated by the Swain–Lupton parameters quantifying these two effects [26] . The calculations indicate in all cases that the transitions are predominantly HOMO-to-LUMO in character. The trends in the electrochemical gaps between the half-wave potentials corresponding to molecular oxidation and reduction closely follow those in the experimental and TD-DFT optical transition energies and the DFT HOMO-LUMO gaps ( Table 1 ). The very close correspondence between the values of the experimental optical and electrochemical gaps (rather than merely trends in these values) is not necessarily to be expected, and presumably arises from a fortuitous balancing of the exciton binding energy stabilizing the excited state and strong solvation of the relatively small ions formed on oxidation or reduction. Accordingly, we have examined the frontier molecular orbitals to explain the origin of the unexpected large redshifts observed in the spectra of the azaacenes on halogenation. The LUMOs of all four compounds are similar in appearance ( Fig. 4a ), explaining the consistent effect of halogenation. In contrast, the geometric shape of the HOMOs differs between the two classes of molecule; 11a ′/ 11b ′ show smaller orbital coefficients on rings 3 and 4 ( Fig. 4a ), whereas in pair 16a/16b the HOMOs have roughly similar coefficients on all rings. The smaller HOMO coefficients on rings 3 and 4 in 11b′ lead to its diminished stabilization by the four chlorine substituents when compared with the pair 16a,b , in which the HOMO coefficients are larger on these rings ( Fig. 4a ). The diminished stabilization of the HOMO when going from 11a′ to 11b′ is the reason for the induced redshift in the diazaacenes. The same effect is also operative for the larger diazapentacenes 15a and 15b , where identical effects are observed according to calculations ( 15a ′, 15b ′), electrochemistry and optical spectroscopy ( Table 1 ). If the proposed explanation is correct, stronger acceptors such as cyano ( 16c ) might be anticipated to have a larger effect and reduce the energy of the optical transitions (and the band gap) further. In such compounds DFT indicates that the HOMO has much smaller coefficients on rings 3 and 4 ( Fig. 4b ). A disjoint orbital structure [19] , that is, spatially separated frontier molecular orbitals results. The disjointing effect is further amplified by electronegative substituents and decreases the transition energies for diazaacenes. When the calculated transition energy for 16c is compared to that for the parent 11c′ (R=H, X=CN), there is a decrease of almost 0.7 eV. This effect is less observed in acenes that have more congruent frontier molecular orbitals [19] . When comparing the tetracene 16a with cyano-substituted 16c , there also occurs a lowering of the computed transition energy; however, the shift of 0.55 eV is smaller than the effect observed when going from 11a ′ to 11c ′. The disjoint frontier molecular orbitals in diazaacenes are the defining features and open the door to amplified substituent effects in the engineering of their electronic and optical properties. N -Heteroacenes in which optical absorption and electron affinity can be tuned independently are within reach. Some of these materials might prove to be promising electron-transport materials. In conclusion, we have prepared the hitherto unknown halogenated azaacenes 11b and 15b,c , which show bathochromically shifted absorptions when compared with their non-halogenated congeners 11a and the previously unknown 15a . Bathochromic shift on chlorination is not observed in the acene/tetrachloroacene series, indicating that the pyrazines are a necessary ingredient for this engineering of optical properties. Quantum chemical calculations reveal that this difference in behaviour can be attributed to the substituent-induced disjoint frontier molecular orbitals of the azaacenes. The interplay between pyrazines and electronegative substituents serves as a uniquely useful tool to manipulate the absorption characteristics of N -heteroacenes. This effect will enhance the design and tuning of acene-type materials for organic electronics and other applications. Synthesis of diazatetracene 11b 1,2,3,4-Tetrachloro-6,11- bis ((triisopropylsilyl)ethynyl)benzo[ b ]phenazine 11b . In ethanol (10 ml) and acetic acid (3 ml), 9 (0.200 g, 3.85 × 10 −4 mol) and 10b (0.0950 g, 3.85 × 10 −4 mol) were heated to reflux overnight. Aqueous workup, filtration washing with cold methanol (10 ml) and column chromatography (10:1, hexane/dichloromethane) give 11b as green-black crystals (0.190 g, 67.6%). mp=179°C (decomp); 1 H-NMR (400 MHz, CDCl 3 ): δ 8.76 (dd, 3 J =3.2 Hz, 4 J =6.8 Hz, 2H), 7.70 (dd, 3 J =3.2 Hz, 4 J =6.8 Hz, 2 H), 1.29-1.27 (m, broad, 42H); 13 C-NMR (80 MHz, CDCl 3 ): δ 140.5, 139.3, 136.6, 134.6, 132.3, 129.0, 127.8, 121.4, 109.7, 101.9, 18.9, 11.6; infrared (KBr): 3,116, 3,062, 2,939, 2,889, 2,862, 2,754, 2,723, 2,360, 2,129, 1,461 cm −1 ; HRMS ( m / z ): [M + ] calcd for C 38 H 46 Cl 4 N 2 Si 2 , 726.19537; found 726.19656; analysis (calcd, found for C 38 H 46 Cl 4 N 2 Si 2 ) C (62.63, 62.60); H (6.36, 6.44). Synthesis of diazapentacenes 15 1,4- Bis ((triisopropylsilyl)ethynyl)anthracene-2,3-diamine ( 13 ). To an oven-dried 1 l Schlenk flask was added 12 (ref. 2 ) (5.20 g, 8.71 × 10 −3 mol) and dry THF (100 ml). After cooling to 0 °C under N 2 , LiAlH 4 (3.31 g, 8.71 × 0 −2 mol) was added over 1 h. After 12 h under inert gas, aqueous workup and column chromatography (3:1, hexane/dichloromethane) gave 13 (4.41 g, 89%). mp: stable to 250°C; 1 H-NMR (400 MHz, CDCl 3 ): δ 8.60 (s, 2H), 7.91 (dd, 3 J =3.2, 4 J =6.4 Hz, 2 H), 7.39 (dd, 3 J =3.2, 4 J =6.4 Hz, 2H), 4.49 (s, 4H), 1.25 (s, 42H); 13 C-NMR (80 MHz, CDCl 3 ): δ 139.7, 130.9, 127.8, 127.5, 124.6, 122.8, 102.8, 102.1, 101.7, 18.7, 11.3; infrared (KBr): 3,047, 2,962, 2,862, 2,719, 2,136, 1,932, 1,913, 1,620, 1,550, 1,539 cm −1 ; HRMS ( m / z ): [M + ] calcd for C 36 H 52 N 2 Si 2 , 568.36691; found, 568.36863. 6,13- Bis ((triisopropylsilyl)ethynyl)-5,14-dihydronaphtho[2,3-b]phenazine ( 14a ). In dichloromethane (50 ml) and acetic acid (3 ml), 13 (0.435 g, 7.65 × 10 −4 mol) and 10a 1 (0.245 g, 2.29 × 10 −3 mol) were heated to reflux for 12 h to give 14a as a metallic red-green solid after aqueous workup and chromatography (hexane) (0.0853 g, 17.5%). mp: 263°C (decomp); 1 H-NMR (400 MHz, CDCl 3 ): δ 8.169 (s, 2 H), 7.75 (dd, 3 J=3.2 Hz, 4 J=6.3 Hz, 2 H), 7.30 (dd, 3 J=3.2 Hz, 4 J=6.4 Hz, 2 H), 6.64 (dd, 3 J=3.3 Hz, 4 J=5.7 Hz, 2 H), 6.33 (dd, 3 J=3.4 Hz, 4 J=5.6 Hz, 2 H), 6.61 (s, 2 H), 1.25 (s, 42 H); 13 C-NMR (80 MHz, CDCl 3 ): δ 136.3, 131.6, 129.1, 128.46, 127.7, 124.8, 122.2, 122.1, 113.0, 103.5, 100.9, 96.0, 18.9, 11.4; infrared (KBr): 3,055, 3,028, 2,956, 2,923, 2,864, 2,752, 2,721, 2,360, 2,198, 2,135, 2,030, 1,870, 1,737 cm −1 ; HRMS ( m / z ): [M + ] calcd for C 42 H 54 N 2 Si 2 : 642.3826; found, 642.3849. 6,13- Bis (triisopropylsilyl)ethynyl)naptho[2,3-b]phenazine ( 15a ). In dichloro-methane (25 ml) 14a (0.100 g, 1.56 × 10 −4 mol) was stirred for 4 h with an excess of MnO 2 ; 15a is obtained after removal of solvent and column chromatography (3:1, hexane : dichloromethane, green solid 0.0995 g, 99%). mp: 265°C (decomp); 1 H-NMR (400 MHz, CDCl 3 ): δ 9.41 (s, 2H), 8.16 (dd, 3 J =3.4 Hz, 4 J =6.9 Hz, 2H), 8.02 (dd, 3 J =3.2 Hz, 4 J =6.6 Hz, 2H), 7.75 (dd, 3 J =3.4 Hz, 4 J =6.9 Hz, 2H), 7.46 (dd, 3 J =3.2 Hz, 4 J =6.6 Hz, 2H), 1.36-1.35 (m, broad, 42H); (80 MHz, CDCl 3 ): δ 145.0, 141.0, 132.9, 132.6, 131.2, 130.5, 128.7, 126.8, 126.8, 120.8, 109.5, 103.8, 19.0, 11.7; infrared (KBr): 3,047, 3,024, 2,956, 2,939, 2,923, 2,862, 2,752, 2,721, 2,136, 2,111, 1,731, 1,600 cm −1 ; HRMS ( m / z ): [M + ] calcd for C 42 H 52 N 2 Si 2 : 640.3669 found 640.3674; analysis (calcd, found for C 42 H 52 N 2 Si 2 ) C (78.69, 78.11); H (8.18, 8.14). 1,2,3,4-Tetrachloro-6,13- bis ((triisopropylsilyl)ethynyl)-5,14-dihydronaphtho[2,3,b]phenazine ( 14b ). In ethanol (3 ml) and acetic acid (1.5 ml), 13 (0.200 g, 3.52 × 10 −4 mol) and 10b (0.0864 g, 3.52 × 10 −4 mol) were reacted under microwave irradiation (120°C, 10 min). After aqueous workup, 14b was purified by column chromatography (9:1, hexane/dichloromethane; metallic red-green solid, 0.0631 g, 23%). mp: stable up to 350°C; 1 H-NMR (400 MHz, CDCl 3 ): δ 8.34 (s, 2H), 7.81 (dd, 3 J =3.2 4 J =6.4 Hz, 2H), 7.39 (dd, 3 J =3.2, 4 J=6.4 Hz, 2 H), 7.18 (s, 2 H), 1.27-1.25 (m, broad, 42 H); 13 C-NMR (80 MHz, CDCl 3 ): δ 133.3, 131.9, 128.3, 127.84, 126.9, 125.5, 123.6, 123.2, 114.9, 105.4, 99.5, 99.1, 18.9, 11.4; infrared (KBr): 3,048, 2,927, 2,918, 2,891, 2,863, 2,853, 2,722, 2,554, 2,129, 1,928, 1,888, 1,797, 1,750, 1,579, 1,553, 1,488, cm −1 ; HRMS ( m / z ): [M + ] calcd for C 42 H 50 N 2 Si 2 Cl 4 : 778.22667; found, 778.22852. 1,2,3,4-Tetrachloro-6,13- bis ((triisopropylsilyl)ethynyl)naphtho[2,3-b]phen-azine ( 15b ). In dichloromethane (25 ml) 14b (0.0631 g, 8.08 × 10 −5 mol) was stirred for 4 h with an excess of activated MnO 2 ; 15b was obtained after removal of solvent and column chromatography (3:1, hexane/dichloromethane; dark-green solid, 0.061 g, 99%). mp: 243°C; 1 H-NMR (400 MHz, CDCl 3 ): δ 9.45 (s, 2H), 8.05 (dd, 3 J =3.1 Hz, 4 J =6.6 Hz, 2H), 7.56 (dd, 3 J =3.1 Hz, 4 J =6.6, 2H), 1.35–1.33 (m, broad, 42H); 13 C-NMR (80 MHz, CDCl 3 ): δ 139.9, 139.4, 134.6, 133.5, 133.5, 132.3, 128.7, 127.4, 127.2, 121.4, 111.1, 102.9, 19.0, 11.6; infrared (KBr): 3,068, 3,045, 2,953, 2,940, 2,926, 2,920, 2,889, 2,863, 2,756, 2,722, 2,136 cm −1 ; HRMS ( m / z ): [M + ] calcd for C 42 H 48 N 2 Si 2 Cl 4 , 776.21102; found, 776.21004; analysis (calcd, found for C 42 H 48 N 2 Si 2 Cl 4 ) C (64.77, 64.56); H (6.21, 6.55). 1,2,3,4-Tetrabromo-6,13- bis ((triisopropylsilyl)ethynyl)-5,14-dihydronaphtho[2,3,b]phenazine ( 14c ). In ethanol (5 ml) and acetic acid (1.5 ml) 13 (0.073 g, 1.28 × 10 −4 mol) and 10c (0.0544 g, 1.28 × 10 −4 ) were refluxed for 12 h. After aqueous workup, 14c was purified by column chromatography (hexane; dark red-green solid, 0.0172 g, 14%). mp: 275 °C (decomp); 1 H-NMR (400 MHz, CDCl 3 ): δ 8.30 (s, 2H), 7.75 (dd, 3 J =3.4 Hz, 4 J =6.4 Hz, 2H), 7.34 (dd, 3 J =3.1 Hz, 4 J =6.4 Hz, 2H), 7.27 (s, 2H), 1.23–1.22 (m, broad, 42H); 13 C-NMR (80 MHz, CDCl 3 ): δ 133.8, 131.9, 128.8, 128.5, 127.8, 125.5, 123.2, 118.4, 109.1, 105.4, 99.6, 98.9, 18.9, 11.4; infrared (KBr): 3,045, 2,939, 2,926, 2,920, 2,887, 2,862, 2,721, 2,534, 2,360, 2,143, 2,127, 1,580 cm −1 ; HRMS ( m / z ): [M + ] calcd for C 42 H 50 N 2 Si 2 Br 4 , 954.02460; found, 954.02184. 1,2,3,4-Tetrabromo-6,13-bis((triisopropylsilyl)ethynyl)naphtho[2,3-b]phenazine ( 15c ). In dichloromethane (25 ml) 14c (0.0172 g, 1.79 × 10 −5 ) was stirred for 4 h with an excess of MnO 2 ; 15c was obtained after solvent removal and column chromatography (3:1, hexane/DCM; dark-green solid; 0.0171 g, 100%). mp: 275°C (decomp); 1 H-NMR (400 MHz, CDCl 3 ): δ 9.46 (s, 2H), 7.99 (dd, 3 J =3.2 Hz, 4 J =6.5 Hz, 2H), 7.50 (dd, 3 J =3.2 Hz, 4 J =6.7 Hz, 2H), 1.34-1.33 (m, broad, 42 H); 13 C-NMR (80 MHz, CDCl 3 ): δ 140.52, 140.48, 133.63, 133.55, 131.7, 129.1, 128.8, 127.45, 127.3, 121.3, 111.1, 103.1, 19.0, 11.7; infrared (KBr) 3,045, 2,954, 2,939, 2,925, 2,889, 2,861, 2,753, 2,722, 2,143, 2,125, 1,531, cm −1 ; ESI ( m / z ): [M + ] calcd for C 42 H 48 N 2 Si 2 Br 4 : 952; found, 952. Correct isotopic splitting pattern. Computational methods Electronic structure computations were performed at the DFT level using the three-parameter hybrid exchange functional from Becke [27] and the correlation functional from Lee et al. [28] (B3LYP). All computations were carried out with a 6-311+G*Pople basis set with the Gaussian 2009 program [28] , [29] . Geometries of the ground singlet states were completely optimized (RMS gradient 3 × 10 −4 , RMS displacement 1.2 × 10 −3 ). Vertical and adiabatic ionization potentials were computed from the unrestricted B3LYP computations of the corresponding ionic states. Vertical and adiabatic excitation energies were computed within the time-dependent (TD)-DFT approach. The first excited electronic state was completely optimized at the TD-DFT level. The totality of the theoretical characterizations (vertical and adiabatic ionization potentials, electron affinities and excitation energies) along with the B3LYP/6-311+G*-optimized geometries for the ground state is included as Supplementary Data . How to cite this article: Appleton A. L., et al. Effects of electronegative substitution on the optical and electronic properties of acenes and diazaacenes. Nat. Commun. 1:90 doi: 10.1038/ncomms1088 (2010).